Two-dimensional enzyme diffusion in laterally confined DNA monolayers Addressing the effects of confinement and crowding on biomolecular function may provide insight into molecular mechanisms within living organisms, and may promote the development of novel biotechnology tools. Here, using molecular manipulation methods, we investigate restriction enzyme reactions with double-stranded (ds)DNA oligomers confined in relatively large (and flat) brushy matrices of monolayer patches of controlled, variable density. We show that enzymes from the contacting solution cannot access the dsDNAs from the top-matrix interface, and instead enter at the matrix sides to diffuse two-dimensionally in the gap between top- and bottom-matrix interfaces. This is achieved by limiting lateral access with a barrier made of high-density molecules that arrest enzyme diffusion. We put forward, as a possible explanation, a simple and general model that relates these data to the steric hindrance in the matrix, and we briefly discuss the implications and applications of this strikingly new phenomenon. Biological molecules are optimized to carry on their functions within highly crowded and confined compartments within living systems [1] , [2] . In biotechnology of synthetic systems, a current trend is to exploit the possibility of assembling functional biomolecules within prototypical devices in which the levels of crowding and compartmentalization are representative of those of living systems [3] , [4] , [5] , [6] , [7] , [8] , [9] , [10] , [11] , [12] , [13] , [14] , [15] . Little is known about the effect of confinement on the properties and functions of these molecules within such crowded systems [1] , [2] ; thus, novel in vitro approaches can provide key information in aiding future biotechnology developments. The immobilization of dense DNA structures on solid supports, obtained by self-assembly and enzymatic manipulations, holds a central role as a tool for developing miniaturized devices with innovative applications, ranging from biosensing [6] , [7] , [8] , [9] to next-generation information technology [14] , [15] . For example, restriction enzymes that cleave double-stranded (ds)DNA molecules are widely utilized in cloning as well as in a number of DNA-based assays [16] , [17] , [18] because they target very specific dsDNA sites. Moreover, these enzymes have key roles in bacterial cell defence against viruses and other parasitic DNAs [16] , and have the ability to diffuse in one-dimension by sliding on the backbone of long dsDNA filaments during their site-searching process [19] . Recently, we have studied the behaviour of a restriction enzyme reaction ( Dpn II) with dsDNA oligomers packed into relatively large (and flat) surface-bound brushy matrices consisting of patches of monolayer with controlled density [20] . We have followed the action of the enzyme by measuring the height reduction of the dsDNA brush because of cleavage using atomic force microscopy (AFM). We have found that the restriction reaction depends on the DNA density, and have demonstrated the existence of a threshold above which the reaction is inhibited (essentially in a stepwise manner) [20] . This result, which has been later confirmed by other groups [21] , [22] , [23] , suggests that the accessibility of dsDNA molecules in these surface-bound brushy matrices critically depends on the inherent steric hindrance. In this paper, we focus on the possible mechanisms underlying the steric hindrance phenomenon by using AFM and fluorescence imaging. We unequivocally show that confining restriction enzymes within these dense and flat dsDNA matrices has a quantifiable effect on their diffusion mechanism. Specifically, regardless of the DNA sequence used, enzymes diffuse inside a dsDNA matrix between the upper (that is, the dsDNA matrix–liquid) interface and the lower (that is, the dsDNA matrix–surface) interface, which are spaced by a gap of only few nanometres that corresponds to the height of the dsDNA matrix with respect to the surrounding surface. This spatial separation is close to the size of the enzyme molecules and, as a consequence, the enzymes diffuse in two dimensions inside the matrix. Furthermore, according to this mechanism, enzymes gain access at the sides of the dsDNA matrix through an area that is 1,000-fold smaller than the total dsDNA matrix–liquid interface. We explain these results by modelling the steric hindrance on the dsDNA matrix–liquid interface, and propose a semiquantitative, steric hindrance-dependent enzyme access mechanism that is inspired by an established model that describes the diffusion of solutes inside polymer matrices [24] . Restriction enzyme reactions in accessible dsDNA matrices We generate, by nanografting, ( Fig. 1a–c ) [25] , [26] , [27] monolayer patches of 44-bp dsDNA molecules with variable density (dsDNA matrices), within bioresistant alkylthiol self-assembled monolayers (SAMs), on an ultraflat gold surface. Nanografting is a technique in which the AFM tip induces, at selected locations, a substitutional exchange of the molecules of the original SAM matrix with new molecules present in solution (thiol-DNA in our case; Fig. 1a–c ). By simply changing the number of times the tip is overwriting the same area during the nanolithography process, we can fine-tune the molecular density in that area [25] . The topographic height of such dsDNA matrices increases with the dsDNA packing and saturates to the length of dsDNA molecules ( ∼ 15 nm) as they stand vertically in crowded monolayers [25] , [26] , [28] . The dsDNA sequences are designed such that they are cut at half height by a restriction enzyme ( Fig. 1d,e ). We assess the reaction by measuring the dsDNA matrix height before ( Fig. 1d ) and after ( Fig. 1f ) enzyme incubation. To obtain mechanistic insight, we tested the action of different restriction enzymes, namely, Dpn II, Bfa I and Bam HI (see DNA sequences in the Methods section), over dsDNA matrices, as a function of their density. 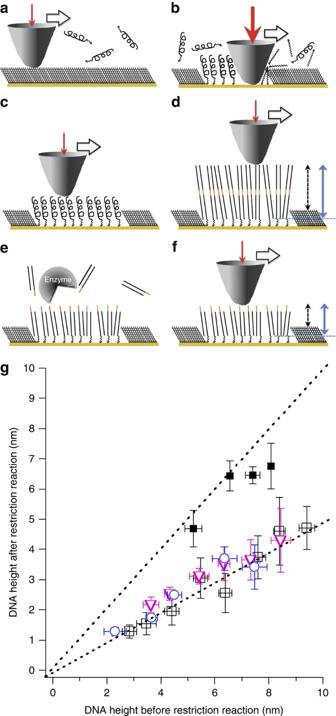Figure 1: AFM detection of restriction enzyme reactions in dsDNA matrices. (a) Schematic view of the DNA nanografting method. An AFM tip contacts an alkylthiol SAM supported by an ultraflat gold surface in the presence of a solution containing a thiol-ssDNA molecule. (b) At high force (∼100 nN), the AFM tip displaces alkylthiol molecules that are replaced by the thiol-ssDNA. (c) The obtained ssDNA matrix can be imaged by AFM at low forces (∼0.2 nN). (d) DNA hybridization follows nanografting to form a dsDNA matrix, in which the dsDNAs have a specific restriction site in the middle (highlighted in orange in the scheme). The absolute initial height (IH) of the dsDNA matrix is determined by AFM imaging at low forces (∼0.2 nN; see blue arrow). This value is derived from the measured relative IH of dsDNA with respect to the surrounding alkylthiol SAM (see dashed black arrow): IH=(relative IH)+(thickness of the alkylthiol SAM)−(length of dsDNA thiol linker) (seeAFM datafor more details in the Methods section). (e) An enzymatic restriction reaction is allowed to occur on the dsDNA matrix. In a successful reaction, dsDNA molecules are cut at half. (f) The absolute final height (FH) of the dsDNA matrix is measured by AFM in the same manner as that for the IH measurement ind(see blue arrow, now shorter). The effect of the reaction on dsDNA matrices is detected by the difference between IH and FH. (g) The plot highlights the effect of three restriction enzyme reactions in the matrices (see DNA sequences in the Methods section) with 2 nm<IH<10 nm,DpnII (open black squares) on Seq1–Seq2 dsDNA,BfaI (open blue circle) on Seq3 dsDNA andBamHI on Seq4 dsDNA (open pink triangles). Patches of Seq3, Seq6 and Seq7 dsDNA are also used withDpnII for control (solid black square). Although for dsDNA with specific affinity for the enzyme FH∼0.5IH, in the control experiment the height remains essentially unchanged. Data are means±s.d. (seeAFM datain the Methods section). Figure 1g shows that, for patches with an average absolute value of initial height (IH) between 2.5 nm and 8 nm (well below saturation), the corresponding absolute average value of the final height (FH) is about half the IH, whereas height stays constant in control matrices, thus indicating a successful (see also Supplementary Fig. S1 ) and specific reaction. We will demonstrate, below, that the mechanism of reaction is similar for three other enzymes. Figure 1: AFM detection of restriction enzyme reactions in dsDNA matrices. ( a ) Schematic view of the DNA nanografting method. An AFM tip contacts an alkylthiol SAM supported by an ultraflat gold surface in the presence of a solution containing a thiol-ssDNA molecule. ( b ) At high force ( ∼ 100 nN), the AFM tip displaces alkylthiol molecules that are replaced by the thiol-ssDNA. ( c ) The obtained ssDNA matrix can be imaged by AFM at low forces ( ∼ 0.2 nN). ( d ) DNA hybridization follows nanografting to form a dsDNA matrix, in which the dsDNAs have a specific restriction site in the middle (highlighted in orange in the scheme). The absolute initial height (IH) of the dsDNA matrix is determined by AFM imaging at low forces ( ∼ 0.2 nN; see blue arrow). This value is derived from the measured relative IH of dsDNA with respect to the surrounding alkylthiol SAM (see dashed black arrow): IH=(relative IH)+(thickness of the alkylthiol SAM)−(length of dsDNA thiol linker) (see AFM data for more details in the Methods section). ( e ) An enzymatic restriction reaction is allowed to occur on the dsDNA matrix. In a successful reaction, dsDNA molecules are cut at half. ( f ) The absolute final height (FH) of the dsDNA matrix is measured by AFM in the same manner as that for the IH measurement in d (see blue arrow, now shorter). The effect of the reaction on dsDNA matrices is detected by the difference between IH and FH. ( g ) The plot highlights the effect of three restriction enzyme reactions in the matrices (see DNA sequences in the Methods section) with 2 nm<IH<10 nm, Dpn II (open black squares) on Seq1–Seq2 dsDNA, Bfa I (open blue circle) on Seq3 dsDNA and Bam HI on Seq4 dsDNA (open pink triangles). Patches of Seq3, Seq6 and Seq7 dsDNA are also used with Dpn II for control (solid black square). Although for dsDNA with specific affinity for the enzyme FH ∼ 0.5IH, in the control experiment the height remains essentially unchanged. Data are means±s.d. (see AFM data in the Methods section). Full size image AFM detection of two-dimensional enzyme diffusion in dsDNA matrices To determine the manner in which restriction enzymes access dsDNA matrices, we engineered substrates consisting of adjacent matrices nanografted with different dsDNA densities. Leaving pH, buffering salts, ionic strength, temperature and enzyme concentration unaltered, we spatially constrained the restriction enzyme reaction. 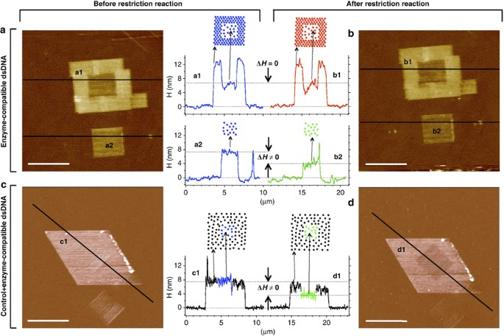Figure 2: AFM detection of 2D enzyme diffusion in dsDNA matrices. Shown is the effect of dsDNA SW density on a restriction enzymatic reaction.aandbare AFM micrographs of two different matrices of Seq1 dsDNA: on the top, a high-density matrix (barrier) surrounds a low-density matrix, whereas at the bottom, the same low-density matrix is grafted without a barrier. Micrographs inaandbwere obtained before and after the enzymatic reaction, respectively. Corresponding line profiles, a1, a2, b1 and b2, are displayed in the centre, together with schematic representations of the DNA density within the matrices. The b1 line profile is in red, and indicates that low-density Seq1 molecules surrounded by the high-density Seq1 barrier remain unchanged after theDpnII reaction. The b2 line profile is in green, and indicates that low-density Seq1 molecules are cleaved byDpnII when the barrier is not present. The evidence indicates that theDpnII reaction occurs in the patch only if the DNA density at the SWs is low. AFM micrographscandddepict a low-density Seq1 dsDNA matrix surrounded by a larger low-density, non-DpnII-cleavable (Seq3) matrix, respectively, before and after the enzymatic reaction. Corresponding line profiles c1 and d1 are displayed in the centre, together with schematic representations of the DNA density in the matrices. Blue and black in c1 refer to Seq1 and Seq3 dsDNA molecules, respectively. In d1, Seq1 molecules are cleaved byDpnII (profile in green). In turn, enzyme molecules diffuse two-dimensionally within the inert low-density dsDNA matrix and retain their enzymatic activity. Graphical schemes represent the DNA density underlying topographic profiles. Scale bar, 3 μm. The topographic AFM images in Figure 2a,b show two distinct but nevertheless identical matrices of low-density Dpn II-cleavable dsDNA (Seq1) molecules before and after the enzymatic reaction, respectively. The structure in the top figure is surrounded by a nanografted high-density Seq1 barrier. The barrier has a relative initial height (IH R )=13 nm with respect to the 'carpet' SAM, whereas in the central area the IH R =7 nm, as shown in the line profile in Figure 2a1 . The matrix in the bottom figure, surrounded by no barrier, has IH R =7.5 nm (that is, the same within the errors as the first patch; Fig. 2a2 ). All heights are calculated from the top of the 'carpet' SAM. To obtain the absolute height of dsDNA in each of these matrices, we add the height of dsDNA buried in the SAM itself, which is ∼ 1.3 nm ( Fig. 1d and Methods section), providing absolute IHs of 14.3 nm, 8.3 nm and 8.8 nm, respectively. From Figure 1g , we expect that dsDNA matrices with an absolute height of <10 nm should be cleaved by the restriction enzyme. The line profiles in Figure 2a,b instead show that the reaction occurs only within the matrix that lacks a surrounding high-density 'fence' structure. This indicates that the access of enzyme to the dsDNA matrix, and therefore the progress of the reaction, strictly depends on the packing of dsDNA molecules at the matrix sides. The same result is observed when the high-density barrier is generated with a control dsDNA sequence (Seq3) lacking the Dpn II restriction site ( Supplementary Fig. S2 and Supplementary Note 1 ). Furthermore, the access inhibition because of the presence of high-density barrier matrices does not substantially depend on their width ( Supplementary Fig. S3 and Supplementary Note 2 ). Thus, we concluded that the Dpn II restriction enzyme cannot access a cleavable dsDNA matrix from its topmost interface with the solution. As a consequence, enzyme access must exclusively occur at the sidewall (SW) of the matrix. Figure 2: AFM detection of 2D enzyme diffusion in dsDNA matrices. Shown is the effect of dsDNA SW density on a restriction enzymatic reaction. a and b are AFM micrographs of two different matrices of Seq1 dsDNA: on the top, a high-density matrix (barrier) surrounds a low-density matrix, whereas at the bottom, the same low-density matrix is grafted without a barrier. Micrographs in a and b were obtained before and after the enzymatic reaction, respectively. Corresponding line profiles, a1, a2, b1 and b2, are displayed in the centre, together with schematic representations of the DNA density within the matrices. The b1 line profile is in red, and indicates that low-density Seq1 molecules surrounded by the high-density Seq1 barrier remain unchanged after the Dpn II reaction. The b2 line profile is in green, and indicates that low-density Seq1 molecules are cleaved by Dpn II when the barrier is not present. The evidence indicates that the Dpn II reaction occurs in the patch only if the DNA density at the SWs is low. AFM micrographs c and d depict a low-density Seq1 dsDNA matrix surrounded by a larger low-density, non- Dpn II-cleavable (Seq3) matrix, respectively, before and after the enzymatic reaction. Corresponding line profiles c1 and d1 are displayed in the centre, together with schematic representations of the DNA density in the matrices. Blue and black in c1 refer to Seq1 and Seq3 dsDNA molecules, respectively. In d1, Seq1 molecules are cleaved by Dpn II (profile in green). In turn, enzyme molecules diffuse two-dimensionally within the inert low-density dsDNA matrix and retain their enzymatic activity. Graphical schemes represent the DNA density underlying topographic profiles. Scale bar, 3 μm. Full size image In general, restriction enzymes specifically recognize nucleotides within the consensus palindromic sequences, thereby enabling phosphodiester hydrolysis [16] , [19] . One possible interpretation of the enzyme access mechanism shown in Figure 2a,b (and Supplementary Fig. S2 ) could be that consensus restriction sites are directly available at the interface, with the solution only on the SWs of the matrix. Therefore, the cleaving reaction would progress from the walls towards the inside. We assessed this hypothesis by nanografting a low-density consensus (Seq1) dsDNA matrix within a larger matrix of control (Seq3) DNA sequence grafted at the same density ( Fig. 2c ). In this set-up, only a non-consensus sequence would be accessible at the SW. The line profile in Figure 2c1 shows that both areas of the patch have IH R =7.5 nm (as for the matrix at the bottom in Fig. 2a ). After the Dpn II reaction ( Fig. 2d1 ), we found that the relative final height (FH R )=4.0 nm in the central matrix, whereas elsewhere, obviously, FH R =IH R . Combined with the data shown in Figure 2a,b (and Supplementary Fig. S2 ), this result demonstrates that Dpn II enzyme molecules can access the consensus (Seq1) dsDNA molecules in the central matrix, after having diffused through a non-consensus (Seq3) low-density dsDNA matrix without cleaving. Inside a non-consensus dsDNA matrix, enzymes diffuse between the upper matrix–liquid interface and the solid substrate at the bottom, which are spaced by a gap of ∼ 9.0 nm (see Figs 2c1, 1d and Methods). Being confined within such a narrow gap, enzyme diffusion in turn becomes two-dimensional (2D). 2D enzyme diffusion in self-assembled dsDNA monolayers To generalize the results shown in Figure 2 , relative to the restriction reaction of Dpn II within low-density dsDNA matrices obtained by nanografting of single-stranded DNAs (ssDNAs), followed by hybridization, we studied the restriction reaction of a different enzyme ( Bam HI) within extended low-density dsDNA monolayers, which were obtained by self-assembly of prehybridized duplexes, formed on the same type of gold substrates. This dsDNA matrix (SAM) was extended on a surface of a few square millimetres, inside of which was nanografted a sole alkylthiol monolayer patch to provide confined sides. 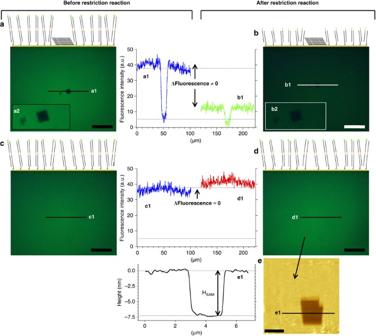Figure 3: The 2D enzyme diffusion in self-assembled dsDNA monolayers detected with fluorescence imaging. (a) A fluorescence image at original magnification ×40 of dsDNA (Seq5) SAM on an ultraflat gold surface. A 10×10-μm2squared patch of bioresistant alkylthiol monolayer is nanografted into the dsDNA SAM. A scheme on the top represents molecules relative to the a1 line profile. (b) The same sample is imaged after a 1-h-long incubation in a solution withBamHI restriction enzyme. The a1 and b1 line profiles in the centre show the fluorescence intensity in arbitrary units surrounding the alkylthiol patch before and after the reaction. The insets a2 and b2 show a digital magnification of the alkylthiol square. The fluorescence intensity decreases by∼70% in the area surrounding the alkylthiol square. The scheme inbrepresents cleaved molecules relative to the b1 line profile. (c,d) Fluorescence images of Seq5 dsDNA forming a homogeneous SAM on an ultraflat gold surface, respectively, before and after 1-h incubation in a solution withBamHI restriction enzyme. Line profiles c1 and d1 show that the reaction does not take place within dsDNA molecules if the alkylthiol square is not generated. This result supports the findings, reported inFigure 2, that is, that enzyme molecules access dsDNA molecules inside the low-density matrix by diffusing from available matrix sides through a vertical gap of few nanometres. (e) The thickness of the unmodified dsDNA monolayer shown indis measured by nanoshaving a 2×3-μm area,∼7.5 nm (see the line profile in e1), which corresponds to an absolute dsDNA height of 6.5 nm (seeFig. 1and Methods). With the values being close to the thickness of low-density dsDNA matrices presented inFigure 2, these dsDNA assemblies likely have the same density. Scale bar ina–d, 50 μm and scale bar ine, 2 μm. In Figure 3 , two SAMs of consensus fluorescently labelled dsDNA (Seq5) with ( Fig. 3a,b ) and without ( Fig. 3c,d ) a nanografted 10×10-ìm 2 patch of a non-fluorescent alkylthiol (see the darker spot in the centre of Fig. 3a ) are imaged before and after the Bam HI reaction. Line profiles in Figure 3a1,b1 indicate that the fluorescence intensity in the area ( ∼ 250×100 μm 2 ) surrounding the alkylthiol patch decreases threefold after the reaction. On the contrary, similar fluorescence line profiles in Figure 3c1–d1 indicate that restriction enzymes cannot cleave the dsDNA molecules in the matrix without the presence of lateral access. The lateral gap available to Bam HI enzymes to access the dsDNA matrix in Figure 3a is quantified in Figure 3d,e in which nanoshaving (see ref. 27 and Methods) was used to measure the thickness of the dsDNA SAM with respect to gold surface, that is, 7.5 nm (see the line profile in Fig. 3e1 ). From the latter, after subtracting the length of the dsDNA thiol linker (see Fig. 1d and Methods), we determined the thickness of the dsDNA matrix to be ∼ 6.5 nm, thus suggesting that the inherent dsDNA density is close to that of the low-density matrices in Figure 2 . In turn, findings shown in Figure 3 generalize the evidence of 2D enzyme diffusion inside dsDNA matrices to different restriction enzymes, and matrices obtained with different self-assembly-based methods. Furthermore, the data presented in Figure 2 (and those presented in Supplementary Fig. S2 and discussed in Supplementary Note 1 ) suggest that the dsDNA density has an important role in the enzyme access mechanism at the matrix sides, and, therefore, in the enzyme 2D diffusion within the matrix. Figure 3: The 2D enzyme diffusion in self-assembled dsDNA monolayers detected with fluorescence imaging. ( a ) A fluorescence image at original magnification ×40 of dsDNA (Seq5) SAM on an ultraflat gold surface. A 10×10-μm 2 squared patch of bioresistant alkylthiol monolayer is nanografted into the dsDNA SAM. A scheme on the top represents molecules relative to the a1 line profile. ( b ) The same sample is imaged after a 1-h-long incubation in a solution with Bam HI restriction enzyme. The a1 and b1 line profiles in the centre show the fluorescence intensity in arbitrary units surrounding the alkylthiol patch before and after the reaction. The insets a2 and b2 show a digital magnification of the alkylthiol square. The fluorescence intensity decreases by ∼ 70% in the area surrounding the alkylthiol square. The scheme in b represents cleaved molecules relative to the b1 line profile. ( c , d ) Fluorescence images of Seq5 dsDNA forming a homogeneous SAM on an ultraflat gold surface, respectively, before and after 1-h incubation in a solution with Bam HI restriction enzyme. Line profiles c1 and d1 show that the reaction does not take place within dsDNA molecules if the alkylthiol square is not generated. This result supports the findings, reported in Figure 2 , that is, that enzyme molecules access dsDNA molecules inside the low-density matrix by diffusing from available matrix sides through a vertical gap of few nanometres. ( e ) The thickness of the unmodified dsDNA monolayer shown in d is measured by nanoshaving a 2×3-μm area, ∼ 7.5 nm (see the line profile in e1), which corresponds to an absolute dsDNA height of 6.5 nm (see Fig. 1 and Methods). With the values being close to the thickness of low-density dsDNA matrices presented in Figure 2 , these dsDNA assemblies likely have the same density. Scale bar in a – d , 50 μm and scale bar in e , 2 μm. Full size image The effect of dsDNA density on restriction enzyme reactions To investigate the access mechanism of enzymes to dsDNA matrices, we next quantified the enzyme reaction as a function of DNA density. 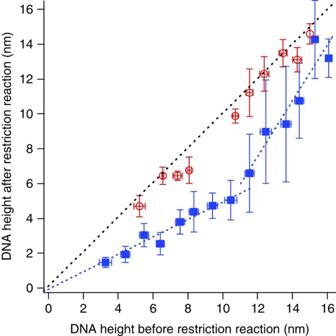Figure 4: The effect of dsDNA density on restriction enzyme reactions inside dsDNA matrices. The plot shows the dispersion of the absolute height of Seq1–Seq2 (blue squares) and control (Seq3, Seq6 and Seq7, open red circles) dsDNA matrices after reaction withDpnII restriction enzyme (FH) versus the initial height (IH). The dashed line in black provides a visual guide for FH=IH (relative to unmodified dsDNA matrices), whereas two fits are shown for the data relative to enzyme-compatible matrices. For IH<12 nm, FH∼0.5IH indicates that these are cleaved. Data are means±s.d. (seeAFM datain Methods section). Figure 4 shows a plot of FH versus IH in the range of patch heights experimentally accessible with AFM. Data were obtained with homogeneous Dpn II-compatible patches (Seq1 and Seq2, blue squares) and control patches (Seq3, Seq6 and Seq7, red circle). Although the control patches on the same surface are not cleaved by the Dpn II enzyme, enzyme-compatible patches are cleaved for IH<12 nm, but remain uncut for IH ⩾ 14 nm. These results confirm that the enzyme diffusion within patches is inhibited in a near stepwise manner for densities higher than a certain critical value, as we found in a previous study [20] , and provide a dsDNA height value of ∼ 13 nm in correspondence to this threshold. Figure 4: The effect of dsDNA density on restriction enzyme reactions inside dsDNA matrices. The plot shows the dispersion of the absolute height of Seq1–Seq2 (blue squares) and control (Seq3, Seq6 and Seq7, open red circles) dsDNA matrices after reaction with Dpn II restriction enzyme (FH) versus the initial height (IH). The dashed line in black provides a visual guide for FH=IH (relative to unmodified dsDNA matrices), whereas two fits are shown for the data relative to enzyme-compatible matrices. For IH<12 nm, FH ∼ 0.5IH indicates that these are cleaved. Data are means±s.d. (see AFM data in Methods section). Full size image Modelling In this section, we propose an explanation of the 2D and density-dependent enzyme diffusion in our surface-bound dsDNA matrices by using simple considerations of inherent steric hindrance. In our experimental conditions, these 44-bp dsDNAs are threefold shorter than the dsDNA persistence length L p ( L ≪ L p ≈50 nm) and are bound to the surface with a very short linker. Thus, the dsDNAs can be modelled as 15-nm-long rigid rods that are free at the topmost end. In this extreme case, the DNA thermal motion can be approximated with the rotational diffusion [29] , [30] , [31] of a rod that is bound at one terminus. The motion of its free terminus is then a random rotation confined on the surface of a hemisphere of radius r = L =15 nm. From the data in Figure 1g and from other data in literature [20] , [25] , [26] , [28] , [32] , it is evident that, for the rod-like dsDNAs, the maximum tilt is limited by the crowding of the DNA as a function of density when an AFM tip contacts the topmost interface of the matrices. Hence, it is likely that the crowding in the matrices limits the rotational diffusion of the dsDNA also in the absence of a contacting object on top, as already derived for a rigid-rod macromolecule in concentrated solution [30] , [31] . In turn, in a very simplified approach, we model that each rod-like dsDNA rotationally diffuses inside a cylinder of volume=π/4· h · d 2 , where h is the matrix height and d is the average distance between two adjacent DNA molecules: the smaller the diameter d of the cylinder, the higher its height h (see the scheme in Fig. 5a,b and ref. 20 ). Because of the dsDNA diffusion anisotropy along the longitudinal section of the cylinder, a dsDNA molecule within our matrices explores a cone inscribed in the above-mentioned cylinder, whereas its free terminus explores a slightly curved surface that can be approximated with the cylinder cross-section. To explain our results, we used this model to account for the steric hindrance exerted near or inside a dsDNA matrix towards slowly diffusing, dilute enzyme molecules. 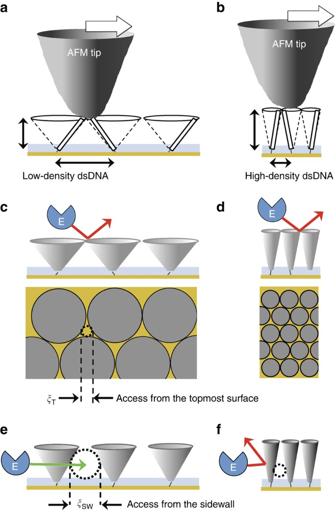Figure 5: Steric hindrance-based model in surface-bound dsDNA matrices underlying 2D enzyme diffusion. (a,b) As shown inFigs 1gand4, the height of the patch (IH), measured while applying a small load with an AFM tip (∼0.2 nN, seeMethodssection), likely depends on the average distance between adjacent dsDNA molecules,d, in the matrices. Here the latter are modelled as rigid rods (lengthL) that are pinned down on the surface and rotationally diffuse, exploring a conic volume. The maximum lateral tilt isθmax=sin−1(2L/d). We expect that the dsDNAs tilt at∼θmaxwhen a force is applied with the AFM tip, and that their measured height is then IH=(L2–d2/4)1/2(seeSupplementary Information Fig. S4). (c,d) The width of the enzyme dimer is close to the diameter of an AFM tip (and the spacing between dsDNA molecules ind). Thus, an enzyme approaching the topmost surface of a matrix is likely hindered to enter the dsDNA matrix, as an AFM tip likewise does not penetrate into the matrix. According to this model and the Peppas description of solutes diffusion in polymeric matrices24, we calculate the hindrance-free mesh widthξ(see dashed circle) in the dsDNA matrix along the direction orthogonal to the surface (ξT, where T stands for top),ξT=0.24·(L2−IH2)1/2. (e,f) Enzyme molecules that approach the monolayer matrix on the SWs can access the matrix volume that is not explored by dsDNAs. Similar to the enzyme top entry, the enzyme top exit is likely hindered by the rotationally diffusing dsDNAs. To calculate the hindrance-free mesh width (see dashed circle) associated with the dsDNA matrix along the direction parallel to the surface (ξSW)24, we modelled the effect of non-negligible, lateral collisions between 2D-diffusing enzyme and dsDNAs inside the matrix by reducing the maximum tilt angle of the latter toθSW=cos−1[(1/θmax)·sin(θmax)] <θmax. In turn,ξSWis defined as the diameter of the circle inscribed between two adjacent rods tilted atθSW(see dashed circle ine). Figure 5: Steric hindrance-based model in surface-bound dsDNA matrices underlying 2D enzyme diffusion. ( a , b ) As shown in Figs 1g and 4 , the height of the patch (IH), measured while applying a small load with an AFM tip ( ∼ 0.2 nN, see Methods section), likely depends on the average distance between adjacent dsDNA molecules, d , in the matrices. Here the latter are modelled as rigid rods (length L ) that are pinned down on the surface and rotationally diffuse, exploring a conic volume. The maximum lateral tilt is θ max =sin −1 (2 L / d ). We expect that the dsDNAs tilt at ∼ θ max when a force is applied with the AFM tip, and that their measured height is then IH=( L 2 – d 2 /4) 1/2 (see Supplementary Information Fig. S4 ). ( c , d ) The width of the enzyme dimer is close to the diameter of an AFM tip (and the spacing between dsDNA molecules in d ). Thus, an enzyme approaching the topmost surface of a matrix is likely hindered to enter the dsDNA matrix, as an AFM tip likewise does not penetrate into the matrix. According to this model and the Peppas description of solutes diffusion in polymeric matrices [24] , we calculate the hindrance-free mesh width ξ (see dashed circle) in the dsDNA matrix along the direction orthogonal to the surface ( ξ T , where T stands for top), ξ T =0.24·( L 2 −IH 2 ) 1/2 . ( e , f ) Enzyme molecules that approach the monolayer matrix on the SWs can access the matrix volume that is not explored by dsDNAs. Similar to the enzyme top entry, the enzyme top exit is likely hindered by the rotationally diffusing dsDNAs. To calculate the hindrance-free mesh width (see dashed circle) associated with the dsDNA matrix along the direction parallel to the surface ( ξ SW ) [24] , we modelled the effect of non-negligible, lateral collisions between 2D-diffusing enzyme and dsDNAs inside the matrix by reducing the maximum tilt angle of the latter to θ SW =cos −1 [(1/ θ max )·sin( θ max )] < θ max . In turn, ξ SW is defined as the diameter of the circle inscribed between two adjacent rods tilted at θ SW (see dashed circle in e ). Full size image Enzyme side entry and 2D diffusion in a dsDNA matrix In our experiments, we used ∼ 20 nM ( ∼ 10 molecules per μm 3 or lower, see Methods section and Supplementary Fig. S1 ) type II restriction enzymes with an approximate size of d E ≈5 nm [16] , [19] , [33] , which are known to form stable homodimers in solutions [16] , and have a diffusion coefficient D enz ≈60 nm 2 μs −1 (ref. 34 ). For low dsDNA densities ( d ≈ L ), a dsDNA likely fully explores the above-mentioned cone in a time τ rod ≈ L 2 D rod −1 , where D rod is the translational diffusion coefficient of the 44-mer dsDNA in solution ( D rod ≈ D enz ) [29] , [30] , [31] , [35] . In our case, we can calculate an exploration time τ rod ≈1–3 μs [31] . In this time interval, the free terminus of each dsDNA rod crosses the (2D) topmost area of this cone several times because of collisions with neighbours. At the same time, dilute enzyme dimers in solution ( ∼ 5 molecules per μm 3 ) in proximity of the dsDNA matrix will explore a volume ∼ L 3 ( ∼ enzyme dimer volume), without colliding with other enzymes and about only once with the top of the matrix. In turn, for each enzyme–dsDNA collision, several dsDNA–dsDNA collisions hinder the enzyme top entry ( Fig. 5c,d ). In view of our model, it is likely that a restriction enzyme dimer, approaching the SW of a dsDNA matrix, has better access to the lower part of the matrix that remains unexplored by the dsDNAs. Once inside the matrix, as opposed to what happens for enzyme approaching the matrix from the top (T), the collisions between the enzymes and the neighbouring rotating dsDNAs likely favour enzyme trapping in the matrix ( Fig. 5e,f ). This model provides a likely qualitative explanation as to why enzyme molecules laterally access and 2D diffuse in a dsDNA matrix. dsDNA density dependence of the 2D enzyme diffusion To account for the results shown in Figure 4 , we next quantified the accessibility of the dsDNA matrices to enzymes using the Peppas model [24] , which is widely used to describe the diffusion of solutes within polymeric matrices. In particular, we calculated the hindrance-free mesh width ( ξ ) as a function of the matrix height IH, associated with the enzyme diffusion in parallel ( ξ SW , solid line in Fig. 6a ), and orthogonal ( ξ T , dashed line in Fig. 6a ) to the surface plane (see dashed circle in Fig. 5c–f , respectively, and Supplementary Fig. S4 ) [24] . Fig. 6b displays the values of FH, previously shown in Figure 4 , renormalized with respect to IH. It is found that, for low-density patches (IH<12 nm), ξ SW is larger than twice of d E (refs 16 , 19 , 33 ) (see Fig. 6a ). In this range, the height of the dsDNA matrix after the enzymatic cleavage is 50% (see Fig. 6b ), and the latter matches with the fact that the enzyme dimers have free access from the SW interface. For high-density patches (IH ⩾ 14 nm), ξ SW becomes smaller than d E (see Fig. 6a ) and, accordingly, the enzymatic cleavage is impeded (see Fig. 6b ). Similarly, enzymatic cleavage is impeded in the entire range of IH , ξ T < d E (see Fig. 6a ), in accordance with the fact that the SW is the most accessible interface. In this model, enzyme diffusion is impeded for matrices higher than the threshold IH ∼ 13 nm, at which the dsDNA density is estimated to be ∼ 5×10 11 molecules per cm 2 (see the Supplementary Fig. S4 ). This value is higher than the estimated dsDNA density in the SAMs shown in Figure 3a,c , which is between 1 and 5×10 11 molecules per cm 2 (see Methods ), according to the Peterson et al . [36] protocol. Therefore, there is agreement between our results and our model on the fact that 2D enzyme diffusion occurs in dsDNA matrices with densities lower than 5×10 11 molecules per cm 2 . Contrary to the predictions of our model in the low-density range, however, it is reasonable to expect that decreasing the dsDNA matrix density would eventually lead to conditions in which the restriction enzyme can directly access a dsDNA matrix from the solution, as the SW and the topmost interfaces would not be distinguishable. Accordingly, data in Supplementary Figure S5 show that Bam HI restriction enzymes have a direct access to the cleavage sites of dsDNA molecules assembled at a sub-monolayer coverage of ∼ 10 10 molecules per cm 2 (see Methods section). This finding suggests that the underlying 2D enzyme diffusion occurs in dsDNA matrices with densities higher than a certain critical threshold (not accounted in our simple model), which is likely between 10 10 and 10 11 molecules per cm 2 . This is currently under investigation in our laboratories. 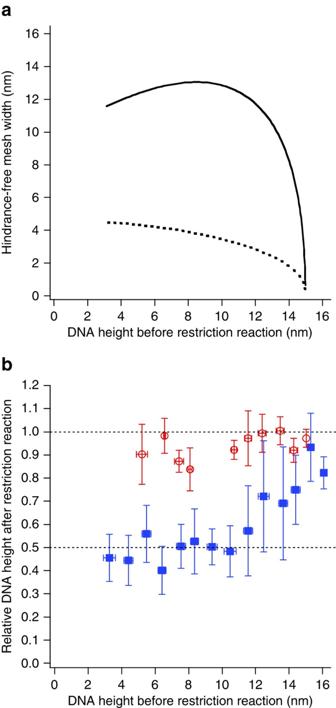Figure 6: Steric hindrance-based model versus experimental results. The panel inaplots the hindrance-free mesh width (ξξ) across the SW, that is, in parallel to the plane,ξSW(solid line) and across the topmost (T) interfaceξT(dashed line), as a function of the initial dsDNA height (IH) according to the model described inFigure 5a–f. The panel inbplots the final dsDNA height (FH)/IH ratio versus IH from the data displayed inFigure 4, relative to theDpnII reaction, for consensus (solid blue squares) and control (open red circles) dsDNA matrices. Data are means±s.d. (seeAFM datain Methods section). For IH<12 nm, the enzymatic cleavage is evident from the fact that FH/IH∼0.5IH (bottom bar in green). In the same range, panelashows thatξSWis bigger than twice the approximate enzyme diameterdEto allow the access of the enzyme dimers. For IH⩾14 nm,ξSWbecomes smaller thandE, whereas, in panelb, the ratio FH/IH is∼1, which means that the enzymatic reaction is impeded (bottom bar in red). On the contrary,ξTis always smaller thandE. These simple calculations suggest that the steric hindrance in the dsDNA matrices is sufficient to explain the experimentally found, dsDNA density-dependent, 2D enzyme diffusion. Figure 6: Steric hindrance-based model versus experimental results. The panel in a plots the hindrance-free mesh width ( ξξ ) across the SW, that is, in parallel to the plane, ξ SW (solid line) and across the topmost (T) interface ξ T (dashed line), as a function of the initial dsDNA height (IH) according to the model described in Figure 5a–f . The panel in b plots the final dsDNA height (FH)/IH ratio versus IH from the data displayed in Figure 4 , relative to the Dpn II reaction, for consensus (solid blue squares) and control (open red circles) dsDNA matrices. Data are means±s.d. (see AFM data in Methods section). For IH<12 nm, the enzymatic cleavage is evident from the fact that FH/IH ∼ 0.5IH (bottom bar in green). In the same range, panel a shows that ξ SW is bigger than twice the approximate enzyme diameter d E to allow the access of the enzyme dimers. For IH ⩾ 14 nm, ξ SW becomes smaller than d E , whereas, in panel b , the ratio FH/IH is ∼ 1, which means that the enzymatic reaction is impeded (bottom bar in red). On the contrary, ξ T is always smaller than d E . These simple calculations suggest that the steric hindrance in the dsDNA matrices is sufficient to explain the experimentally found, dsDNA density-dependent, 2D enzyme diffusion. Full size image By combining an AFM-based molecular nanomanipulation method with AFM imaging and fluorescence microscopy, we have examined the effect of confinement on enzymatic reactions of surface-bound dsDNA matrices. In particular, we have observed a novel effect of confinement on the diffusion of restriction enzymes within laterally confined monolayers of short dsDNA molecules that depends on the dsDNA density. We monitored enzyme diffusion in such matrices by measuring the effects of the enzyme cleavage on the inherent dsDNA molecules. Selectively, the cleavage induces a detectable height decrease of a matrix and/or a loss of fluorescent label on its topmost interface. We have demonstrated that, during a few-hours-long reaction, the access of enzyme molecules in solution through the topmost matrix–liquid interface (top entry) is negligible. Instead, enzyme molecules obtain access from the matrix sides (side entry) with areas having lower orders of magnitude. Once the enzymes enter the DNA matrix, they reach a location of the dsDNA matrix that is distant from the sides. This finding suggests that enzymes are retained within the matrix, and therefore diffuse through it in a 2D manner. In our experiments, however, we cannot determine whether a small but non-negligible top exit can occur for the enzyme, a process compatible with the underlying 2D-diffusion process. In fact, we could only indirectly detect the presence of enzyme molecules within the surface-bound matrix. Direct detection (for example, based on fluorescent (FRET) [37] ) would require enzyme modification, and is beyond the scope of this work. Similarly, top entry cannot be completely excluded, and may increase as a function of enzyme concentration (in these experiments the concentration was ∼ 20 nM, see Methods section) and incubation time, which can favour desorption of dsDNAs and increase the number of surface defects. It is important to note here that enzyme-ready DNA duplexes can be formed either by hybridizing ssDNAs preimmobilized by nanografting or by immobilizing prehybridized duplexes. In general, the former process may lead to an absence (or incomplete formation) of duplexes [11] , [36] , as hybridization efficiency depends on ssDNA density. However, in a previous study, we demonstrated that low-density (<10 12 molecules per cm 2 ) ssDNA matrices produced by nanografting exhibit high hybridization efficiency [20] , [25] , [36] , and furthermore the results obtained in the two conditions are compatible. The side-access effect reported in this study has not been hitherto described, although other investigations demonstrated enzymatic reactions on surface-bound DNA molecules [6] , [21] , [22] , [23] , [38] , [39] , [40] , [41] , [42] , [43] , [44] . These studies used either longer dsDNA molecules [23] , [40] or molecules provided with significantly less-rigid surface linkers and/or different chemical strategies for DNA self-assembly [6] , [23] , [39] , [41] . Several studies involved ligation enzymes [42] , [43] , the reactions of which occurred on DNA-binding sites that are readily available on the topmost interface of the matrices. In contrast, Corn [39] , and Daube and co-workers [40] used restriction enzymes and dsDNA densities close to our experimental conditions, and their results substantially differ from ours, as enzyme top entry was demonstrated. It is possible that the surface roughness in our case was low enough ( ∼ 0.5 nm) to significantly reduce the number of defects in dsDNA matrices, and that higher surface roughness values [40] favour the formation of multiple top-access points. Alternatively, dsDNA molecules with L ∼ L p (or longer), or those provided with longer linkers [39] , [40] , may have significantly reduced collisions with their neighbours [31] , thus increasing the mechanical compressibility of the matrix [25] and, in turn, increasing top-entry accessibility to enzymes. In this work, we have put forward a functional model that relates the hindered enzyme top entry and the density dependence of the 2D enzyme diffusion in a laterally confined matrix of short and, therefore, rigid dsDNA molecules, to steric effects in the matrix. Despite that this semiquantitative model provides a plausible explanation of our findings, and additional effects may (or should) be considered to further extend the implications of our work: the 2D diffusion could be favoured by reversible enzyme absorption on the ethylene-glycol-terminated molecules on the surface near the SW, as suggested by a recent neutron reflectivity study of Schreiber and co-workers [45] . This effect may help increase the enzyme concentration in the area surrounding the matrices (that is, at the matrices sides) and, similarly, the enzymes would be trapped within the matrix while they diffuse two-dimensionally. The above-mentioned work, which was based, however, on protein concentrations much higher than in our case, demonstrates an oscillating protein density profile, right above a protein-depleted hydration layer, adjacent to the top-oligo-ethylene-glycol-3 (TOEG3), which inhibits the protein from unfolding and irreversible bonding. Protein/surface interactions are, in general, complex phenomena that depend on several parameters, including local electrostatic interactions and diffusion [45] . In contrast to Schreiber and co-workers [45] , Grunze and co-workers [46] probed the resistance to protein adsorption on TOEG3 SAMs on gold surfaces by scanning force microscopy using negatively charged and hydrophobic AFM tips to mimic a protein in solution. Their force–distance measurements showed that electrostatic effects are important factors for the interaction of proteins on the TOEG3 on gold, and that this interaction markedly changes on slight changes in the molecular orientation of TOEG3 molecules on different metal surfaces, in a manner that is difficult to account for using a simplified model. The net charge of a DNA matrix is higher than that on our TOEG SAMs [47] , and the abrupt change at the side of our matrices may significantly affect the local surface potentials at the sides. In turn, enzyme side entry and consequent 2D diffusion could be enhanced [16] , [48] . In conclusion, we anticipate that the possibility of confining the diffusion of enzymes, or of proteins in general, inside self-assembled (that is, low cost) nanostructured matrices at the interface with liquids, has important functional implications on the development of new nanofluidic approaches [49] , [50] , [51] to the detection, manipulation and analysis of biological molecules. Preparation of bioresistant ultraflat alkylthiol SAMs About 100-nm-thick gold film is deposited by electron beam evaporation in a vacuum chamber (pressure about 10 −5 mbar) on a freshly cleaved mica sheet (Mica New York, clear ruby muscovite) at a rate of 0.1 nm s −1 . The obtained gold on mica sheet is cut in samples of a few millimetres in size. Silicon samples are cut from a wafer such that they are smaller in size than gold on mica slices (no special purity is required for silicon wafers). A drop of SU8-100 (negative tone photoresist, MicroChem) is dispensed on each gold surface [20] . Each silicon sample is contacted with the glue by its polished surface. Silicon samples are gently pressed to distribute the glue in the interface between the gold and silicon. The glue is cured at 130°C for at least 48 h. Samples are allowed to slowly cool down to room temperature to avoid thermal stresses that can result in the detachment of the gold film from the mica substrate. In turn, the gold surface that is buried in contact with mica remains protected, and samples are stored without any further precaution. An ultraflat gold surface is obtained by mechanically stripping the mica substrate from the silicon-SU8-gold sandwich. A freshly stripped gold surface is immediately dipped and incubated overnight in a 100-μM ethylene-glycol-terminated alkylthiol, that is, HS-(CH 2 ) 11 -(O-CH 2 -CH 2 ) 3 -OH (TOEG3) or HS-(CH 2 ) 11 -(O-CH 2 -CH 2 ) 6 -OH (top-oligo-ethylene-glycol-6, TOEG6) (Prochimia and Sigma Aldrich) solution in pure ethanol (Fluka or Thomas Scientific, purity ⩾ 99.8%). Both obtained alkylthiol SAMs resist the nonspecific adsorption of biomolecules used in our experiments and have AFM-measured roughness of ∼ 0.2 nm over a scanning area of 50×50 μm 2 (refs 45 , 52 ). ssDNA sequences used Thiolated 44-base-long ssDNA molecules containing a recognition sequence of 4–6 bp at half height (specific to the restriction enzymes used) were purchased from Sigma Genosys, Biomers and IDT at HPLC purification (unlabelled complementary sequences not shown): Seq1 :: SH-((CH) 2 ) 6 -5′-CAAAACAGCAGCAATCCAAA GATC AGACACCCGATTACAAATGC-3′; Seq2 :: SH-((CH) 2 ) 6 -5′-AAAAAAAAAAAAAAAA GATC ATGAAGCACATCAGAGTCTCCTAC-3′; Seq3 :: SH-((CH) 2 ) 6 -5′-CAAAACAGCAGCAATCCAAA CTAG AGACACCCGATTACAAATGC-3′; Seq4 :: SH-((CH) 2 ) 6 -5′-CAAAACAGCAGCAATCCAA GGATCC GACACCCGATTACAAATGC-3′; Seq5 :: SH-((CH) 2 ) 6 -5′-CAAAACAGCAGCAATCCAA GGATCC GACACCCGATTACAAATGA-3′; complementary Seq5 :: Alexa488dye-5′-TCATTTGTAATCGGGTGTC GGATCC TTGGATTGCTGCTGTTTTG-3′; Seq6 :: SH-((CH) 2 ) 6 -5′-AAAAAAAAAAAAAAAAAAAAATGAAGCACATCAGAGTCTCCTAC-3′; and Seq7 :: SH-((CH) 2 ) 6 -5′-AAAAAAAAAAAAAAAAGAACATGAAGCACATCAGAGTCTCCTAC-3′. Nanografting of ssDNA matrices AFM experiments were carried out with a MFP-3D-Stand Alone Asylum Research (Asylum Research; 100×100-μm scan size; AFM1), a XE-100 PARK/PSIA System (PARK System; 50×50 μm scan size; AFM2) and a Digital Instruments MultiMode AFM with a Nanoscope IIIa controller (Veeco; 12×12 μm scan size; AFM3). All AFM experiments were carried out in liquid by using commercially available liquid cells. All nanografting experiments are carried out with silicon cantilevers having a spring constant between 0.5 and 1.5 N m −1 (typically MikroMasch, 19-series, spring constant about 0.6 N m −1 , tip radius <10 nm). Nanografting is carried out by applying forces of 80–150 nN and at a tip speed of ∼ 3 μm s −1 . Before nanografting, the liquid cell is filled with the ssDNA containing buffered solution. High-density and low-density DNA matrices can be obtained by nanografting within TOEG3 SAMs from a 3:2 mixture (v/v) of a 10-μM ssDNA, 1-M NaCl solution in TE-buffer (10-mM Tris-HCl, 1-mM EDTA, pH 7.2 at 25°C; Sigma Aldrich) in Milli-Q water (resistivity=18.2 MΩcm) and absolute ethanol (Fluka or Thomas Scientific, purity ⩾ 99.8%) [25] . Furthermore, low-density DNA matrices are also obtained by nanografting within TOEG6 SAMs from a 5- to 10-μM ssDNA and 1-M NaCl solution in TE-buffer (10-mM Tris-HCl, 1-mM EDTA, pH 7.2 @ 25°C; Sigma Aldrich). Hybridization of ssDNA matrices After nanografting, surfaces were copiously washed with the ssDNA-free nanografting solution. Hybridization of DNA matrices was performed by incubating surfaces in 2-μM solutions of complementary DNA in 4-M NaCl TE-buffer (Sigma Aldrich) in Milli-Q water. After hybridization, surfaces were copiously washed with DNA-free 4-M NaCl and 1-M NaCl TE buffers. AFM data The relative topographic height of DNA matrices is measured by AFM in contact mode before and after restriction reactions at a force of ∼ 0.2 nN. The softest silicon cantilevers (typically MikroMasch, 38-series, nominal spring constant 0.03 N m −1 , tip radius <10 nm) are used at a tip speed of ∼ 5 μm s −1 (which may change between different apparatus according to their feedback performances), in NEB*-buffer (100-mM NaCl, 10-mM MgCl 2 , 50-mM Bis-Tris-HCl, pH 6.0 at 25°C (Sigma Aldrich) in Milli-Q water) [20] . The absolute height of dsDNA molecules is H Abs = H Rel + H TOEG n − H C6 , where H Rel is the dsDNA relative height (see Fig. 1d,f ), H TOEG n is the height of the TOEG n alkylthiol SAM ( n =3,6) and H C6 is the length of the dsDNA thiol linker (C6-SH). H TOEG3 =2.3 nm, H TOEG6 =3.1 nm and H C6 =1.0 nm [52] . The roughness (RMS) on the TOEG surfaces was measured as RMS TOEG ∼ 0.2 nm. In turn, on average, H Abs =1.3±0.2 nm for TOEG3 and H Abs =2.1±0.2 nm for TOEG6, in agreement with previous studies [52] . The roughness on the dsDNA surfaces was measured to be 0.2 nm<RMS dsDNA <1 nm. Each value of initial and FH, and their corresponding standard deviations relative to Figures 1g , 4 and Supplementary Figure S1 , were obtained by averaging the calculated absolute heights of (at least) ten different dsDNA patches before and after the enzymatic reaction, respectively. Standard deviations relative to the ratio FH/IH in Figure 6b were derived from data in Figure 4 . In the AFM images shown in Figure 2 , Supplementary Figures S2 and S3 , the surrounding SAM is a TOEG3. In the AFM images discussed in Figure 3 , the nanografted alkylthiol patch is a TOEG6. Data relative to Figures 1 , 4 , 6 and Supplementary Figure S1 are derived from dsDNA matrices nanografted both in TOEG3 and TOEG6. Data relative to Figure 1 were obtained with AFM1-2-3 (see the definitions in 'Nanografting of ssDNA matrices, equipment and settings'); data in Figure 2a,b were obtained with AFM2; data in Figure 2c,d were obtained with AFM1; data in Figure 3e were obtained with AFM3; data in Figure 4 and, thus, Figure 6 were obtained with AFM1-2-3; data in Supplementary Figure S1 were obtained with AFM1-2; data in Supplementary Figures S2a–d and S3a,b were obtained with AFM3; and data in Supplementary Figure S3c and d were obtained with AFM2. AFM profiles shown in Figures 2 , 3 , Supplementary Figure S2 and S3 were obtained by averaging 12 individual line profiles in correspondence to the lines shown in the display. Differential line analysis of the effect of restriction enzyme reactions shown in these figures refers to the same locations of dsDNA matrices as displayed. Ultraflat fluorescently labelled dsDNA SAMs dsDNA molecules are obtained by incubating 1:1 in molar ratio of Seq5-SH and Seq5-Alexa488dye strands for 2 h at 37°C in a 1-M NaCl solution in TE buffer (10-mM Tris-HCl, 1-mM EDTA, pH 7.2 at 25°C in Milli-Q water; Seq5 differs from Seq4 in correspondence to the last nucleotide at the 5′ end for improving the performance of the fluorescent dye). Low-density SAMs of Seq5 dsDNA are prepared on ultraflat gold samples by incubating a preimmobilized gold sample in a 1-μM solution of dsDNA-SH for 2 min. The estimated density is between 1 and 5×10 11 molecules per cm 2 (ref. 36 ). A sub-monolayer dsDNA coverage was obtained by incubating the sample for 20 s, and was estimated to be ∼ 10 10 molecules per cm 2 (ref. 36 ). After incubation, samples are thoroughly rinsed with DNA-free 1-M NaCl TE buffer, pH 7.2. Samples were incubated in 100-μM solution of 1-mercaptohexanol (Sigma Aldrich) in TE buffer (pH 7.2) for 1 h to block the gold surface, thus protecting from the nonspecific adsorption of biomolecules. Samples were again thoroughly rinsed with 1-M NaCl TE buffer, pH 7.2. Nanografting of TOEG6 is performed within the obtained dsDNA SAM in 10-μM TOEG6, 1-M NaCl solution in TE buffer, pH 7.2. All fluorescence microscopy experiments (shown in Fig. 3a–d and Supplementary Fig. S5a,b ) were carried out with a Nikon Eclipse E400 microscope (Nikon) equipped with an Infinity 2 camera. All fluorescence images were acquired with a Blue Excitation Filter Block b-2E/C (excitation filter wavelength: 465–495 nm; dichromatic mirror cutoff wavelength: 505 nm; and barrier filter wavelength: 515–555 nm) at the same optical magnification and intensity exposition to avoid undesired photobleaching effects. Fluorescence intensity profiles shown in Figure 3a–d and Supplementary Figure S5a,b were obtained by averaging 24 individual line profiles. Restriction enzyme reactions The restriction enzymes used in this study are Dpn II, Bam HI and Bfa 1, which were purchased from New England BioLabs and were used with the corresponding reaction buffers supplied by the manufacturer. Reactions were carried out at 0.2 U μl −1 ( ∼ 20 nM) for 3 h (unless otherwise specified). After enzymatic reactions, surfaces were copiously washed with the corresponding enzyme-free reaction buffer, followed by rinsing in NEB*-buffer (100-mM NaCl, 10-mM MgCl 2 , 50-mM Bis-Tris-HCl, 1-mM Dithiothreitol, pH 6.0 at 25°C (Sigma Aldrich) in Milli-Q water) and, subsequently, in 1-M NaCl TE buffer [20] . Data analysis All AFM data were analyzed with the proprietary programs provided with the corresponding AFM apparatus. AFM data were also analyzed with SPIP ( http://www.imagemet.com/ ) and Gwyddion ( http://gwyddion.net/ ). Fluorescence data were analyzed with Image J ( http://rsbweb.nih.gov/ij/ ). All data were processed with Microsoft Excel ( http://office.microsoft.com ) and Igor Pro 6.0 ( http://www.wavemetrics.com/ ). All the colour scales used for the AFM displays of this work are linear. How to cite this article: Castronovo, M. et al . Two-dimensional enzyme diffusion in laterally confined DNA monolayers. Nat. Commun. 2:297 doi: 10.1038/ncomms1296 (2011).